Regional insight into savanna hydrogeomorphology from termite mounds Global vegetation models predict the spread of woody vegetation in African savannas and grasslands under future climate scenarios, but they operate too broadly to consider hillslope-scale variations in tree–grass distribution. Topographically linked hydrology–soil–vegetation sequences, or catenas, underpin a variety of ecological processes in savannas, including responses to climate change. In this study, we explore the three-dimensional structure of hillslopes and vegetation, using high-resolution airborne LiDAR (Light Detection And Ranging), to understand the long-term effects of mean annual precipitation (MAP) on catena pattern. Our results reveal that the presence and position of hillslope hydrological boundaries, or seeplines, vary as a function of MAP through its long-term influence on clay redistribution. We suggest that changes in climate will differentially alter the structure of savannas through hydrological changes to the seasonally saturated grasslands downslope of seeplines. The mechanisms underlying future woody encroachment are not simply physiological responses to elevated temperatures and CO 2 levels but also involve hydrogeomorphological processes at the hillslope scale. The spatial distribution of vegetation has ecological consequences for landscapes [1] , and is considered key to maintaining ecological functioning and preventing catastrophic shifts in ecosystems [2] . In savannas, the relative distribution and patterns among woody and herbaceous vegetation has drawn much scientific attention [3] , [4] , as the balance between these growth forms profoundly influences ecosystem function [5] , [6] . Not surprisingly, much of the discussion has centred on the regional-scale climatic/ecological controls that define savanna boundaries with other biomes, as opposed to the within-savanna, catena-scale heterogeneity [7] . Catenas exhibit clear shifts in vegetation structure and composition from hillslope crest to valley bottom, reflecting changes in underlying soil and hydrological conditions [8] , [9] . Accumulation of clay in valley bottoms and lower slope positions leads to the emergence of seeplines [10] , where water moving downslope through soil backs up against the clay-enriched zone. Seeplines form boundaries between broad-leafed woody savanna (upslope) and grassland (downslope), where seasonally waterlogged soils preclude the establishment and persistence of trees [7] . These different catena elements provide a diverse array of resources and habitat for organisms [11] , and exhibit differential rates of nutrient cycling [10] . Traditional explorations of catenas have taken place over limited two-dimensional (2D) geographical extents on select hillslopes (plan or profile view) because we lacked the imaging and computing power to develop the regional 3D perspective needed to understand the catena processes that structure savanna communities. We conducted a high-resolution 3D assessment of savanna landscapes, incorporating not only terrain morphology and vegetation structure but also the structure and distribution of termite mounds, across a regional (250 km) precipitation gradient. Termite mounds are conspicuous features of savannas [12] ; however, although their self-organizing spatial arrangements have attracted much interest [13] , [14] , the ecological insight that their landscape distribution could provide has received less focus. Mound-building termites, such as the Macrotermes , predominantly build their nests on well-drained soils to avoid inundation, but need readily available clays for mound construction [15] , [16] . These habitat requirements could render them as useful indicators of hydrogeomorphic conditions; too much clay should prevent mound establishment because of slow permeability and increased periods of inundation, and too little clay should preclude or limit mound construction. In this study, we evaluated the density, size–class distribution and hillslope distribution of 41,227 termite mounds ( Macrotermes ) across 50,000 ha of semiarid granitic savanna in Kruger National Park, South Africa, an area minimally affected by human-dominated land use. We also explored the horizontal and vertical structure of all woody plants within the study area. All measurements were derived from the Carnegie Airborne Observatory (CAO), an integrated Light Detection And Ranging (LiDAR) and hyperspectral remote-sensing system [17] , and were recorded at 1.12 m resolution. Our analyses spanned a mean annual precipitation (MAP) gradient of 450–750 mm, positioning the study within the realm of 'climatically determined savannas' (<650 ± 134 mm MAP) [18] , [19] . We found termite mounds to be tightly coupled with the soil and hydrological characteristics of the hillslopes. Mounds were distributed across the entire hillslope under driest conditions, but were restricted to crest locations at the intermediate and wetter sites where catena patterns were strongly expressed; that is, the hillslope was well differentiated into its different catena elements of woodland, seepline and grassland. We used the downslope limit of mounds to delineate the seepline and found that its hillslope location varied as a function of MAP. Future changes in climate are likely to drive differential responses in savanna landscapes given the diversity of catena expression under different MAP. Vegetation responses to climate are not only physiological but involve hydrological processes at the hillslope scale. Broad variation in vegetation and termite mound structure The CAO enabled a detailed exploration of the savanna vegetation and landscape structure in both vertical ( Fig. 1a ) and horizontal ( Fig. 1b ) dimensions. The ability of the CAO LiDAR component to penetrate vegetation and map termite mounds provided one of the clearest illustrations of regular pattern formation observed in nature ( Fig. 1c ). Below 650 mm, we expected maximum woody cover to be constrained by, and increase linearly with, MAP [19] . However, the mean woody cover in our study region decreased with increasing MAP ( Fig. 2a ), and is therefore more variable in its response to precipitation than is maximum cover. Termite mound density was uncorrelated with MAP, and was lowest towards the middle of the gradient ( Fig. 2a ). For analysis purposes, we divided the gradient into three core zones (dry, intermediate and wet), which contained similar woody vegetation and termite mound properties ( Fig. 2a ). Woody height–class distributions differed significantly between the three MAP zones, and shifted from a shrub-dominated landscape with few tall trees to a more homogenous distribution of canopy height, with increasing precipitation ( Fig. 2b ). Canopy height distribution under intermediate MAP closely resembled the average of the wetter and drier zones. Although we found the highest woody cover in the driest zone (32%), structural analyses showed that half of this cover is contained in the shrub layer (<2 m tall). Therefore, the absence of a positive relationship between mean woody cover and MAP ( Fig. 2a ) partly stems from structural variation in vegetation across the gradient, and also reflects differences in the hillslope distribution of broad-leafed savanna and grassland. Termite mounds were taller on an average in the intermediate MAP zone (1.6 ± 0.5 m) than in drier (1.2 ± 0.4 m) and wetter (1.0 ± 0.3 m) zones. The size–class distribution of mounds also differed across the gradient, with small mounds (~1 m) dominating the wetter zone, whereas the other zones, and the intermediate in particular, supported a greater proportion of taller mounds ( Fig. 2c ). 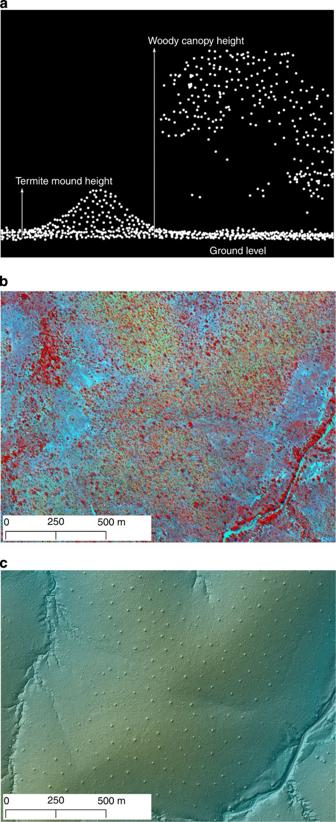Figure 1: A 3D measurement of savanna structure with the Carnegie Airborne Observatory (CAO). (a) Cross-section through the LiDAR point cloud illustrating the determination of ground level elevation, termite mound height and woody vegetation canopy height. (b) Spatial representation of photosynthetically active savanna vegetation (red). (c) Hillshade view of savanna terrain, revealing the prominence and regulated spacing of termite mounds across the landscape. Figure 1: A 3D measurement of savanna structure with the Carnegie Airborne Observatory (CAO). ( a ) Cross-section through the LiDAR point cloud illustrating the determination of ground level elevation, termite mound height and woody vegetation canopy height. ( b ) Spatial representation of photosynthetically active savanna vegetation (red). ( c ) Hillshade view of savanna terrain, revealing the prominence and regulated spacing of termite mounds across the landscape. 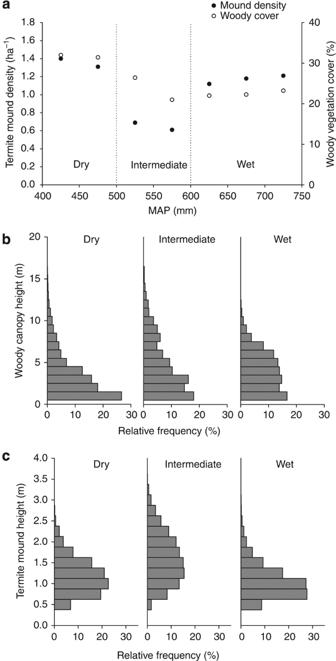Figure 2: Broad-scale variation in termite mound and woody vegetation as a function of mean annual precipitation (MAP). (a) Termite mound density was uncorrelated with MAP (r2=0.01;P=0.82;n=7), but percentage woody cover decreased with increasing MAP (r2=0.61;P=0.02;n=7). Three core MAP zones (dry, intermediate and wet) were delineated on the basis of mound density and percentage woody cover. (b) Height-class distribution of woody vegetation differed among all three MAP zones (Kolmogorov–Smirnov test;P<0.001;n=10,000). (c) Size-class distribution of termite mounds differed among all three MAP zones (Kolmogorov–Smirnov test;P<0.001;n=5,000). Full size image Figure 2: Broad-scale variation in termite mound and woody vegetation as a function of mean annual precipitation (MAP). ( a ) Termite mound density was uncorrelated with MAP ( r 2 =0.01; P =0.82; n =7), but percentage woody cover decreased with increasing MAP ( r 2 =0.61; P =0.02; n =7). Three core MAP zones (dry, intermediate and wet) were delineated on the basis of mound density and percentage woody cover. ( b ) Height-class distribution of woody vegetation differed among all three MAP zones (Kolmogorov–Smirnov test; P <0.001; n =10,000). ( c ) Size-class distribution of termite mounds differed among all three MAP zones (Kolmogorov–Smirnov test; P <0.001; n =5,000). Full size image Hydrogeomorphic controls at the hillslope scale Termite mounds were not uniformly distributed across the landscape, but occurred more frequently in elevated hillslope positions ( Fig. 3a ). The downslope limit to termite mound distribution followed contours of elevation above river channels ( Fig. 3b ), highlighting the importance of hydrogeomorphology in shaping their distribution. The boundary in termite mound distribution demarcated the catena seepline, the hillslope position where broad-leafed savanna on sandy soils transitions to grassland on clayeyer soils ( Fig. 3c ). Quadrat-based analyses showed that hillslope boundaries in termite mound density coincided with the broad-leafed savanna/grassland divide in both intermediate and wetter zones, as woody vegetation upslope of the seepline boundary was significantly greater than that at the downslope of the seepline (paired t -test; P <0.001, n =100). The seepline was situated further from river channels and was more distinct in the intermediate zone (62% difference in woody cover between grassland and broad-leafed savanna) than in the wetter zone (28% difference in woody cover). No broad-leafed-savanna/grassland divide was identifiable in the drier zone, where the riparian corridor transitioned directly to broad-leafed vegetation. 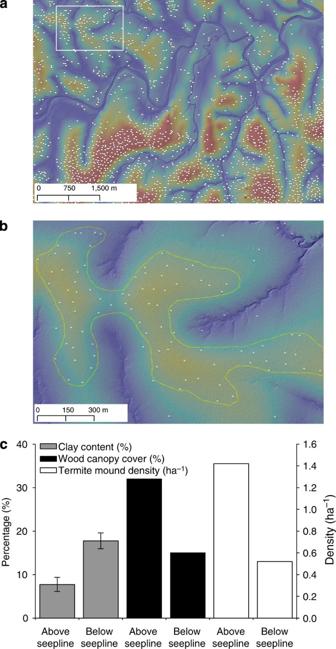Figure 3: Landscape distribution of termite mounds demarcate the catena hillslope seepline. (a) Hillshade view of a subset of the intermediate MAP landscape. Warm colours represent higher elevations above river channels, and white dots indicate termite mound locations. (b) The downslope limit of termite mound distribution demarcates the catena seepline, shown in yellow. (c) Differences in clay content (n=30 surface samples; error bars are 2 s.e.), percentage woody vegetation cover and termite mound density on either side of the seepline. Figure 3: Landscape distribution of termite mounds demarcate the catena hillslope seepline. ( a ) Hillshade view of a subset of the intermediate MAP landscape. Warm colours represent higher elevations above river channels, and white dots indicate termite mound locations. ( b ) The downslope limit of termite mound distribution demarcates the catena seepline, shown in yellow. ( c ) Differences in clay content ( n =30 surface samples; error bars are 2 s.e. ), percentage woody vegetation cover and termite mound density on either side of the seepline. Full size image Hillslope-scale heterogeneity across precipitation gradients Hillslope-scale patterns of woody vegetation cover and termite mound density varied across the precipitation gradient, with the wetter and drier zones being most dissimilar, and the intermediate zone sharing the characteristics of both ( Fig. 4 ). Woody canopy cover was highest in riparian corridors of drier and intermediate zones (30–40%), but decreased with distance from river channels. Moving further away from river channels, woody cover then remained constant across the hillslopes of the drier zone ( Fig. 4a ), but increased again with distance from the river channel in the intermediate ( Fig. 4b ) and wetter zones ( Fig. 4c ). The hillslope pattern under drier MAP deviated from the catena model as no grassland was evident ( Fig. 4a ), but catenas were strongly expressed in intermediate ( Fig. 4b ) and wetter zones ( Fig. 4c ). Outside the riparian corridor, woody cover increased consistently with distance from the river in the wetter zone, but unlike the drier and intermediate zones, termite mound density decreased towards the top of the hillslope ( Fig. 4c ). This pattern suggests that the soils of some crests are too sandy to support the construction of mounds, and highlights the value of considering not only 3D vegetation structure, but also mound structure and spatial pattern. These hillslope signals were captured in the composite landscape representations of mound density and woody cover ( Fig. 4 ), despite the variability associated with differing hillslope curvatures, lengths, aspects and elevations above river channels. Although the patterns were most clearly defined on individual hillslopes within each site (for example, colour inserts Fig. 4 ), it is remarkable that the integrated averages of entire 3D landscapes in each setting still reflected the fundamental hillslope-scale trends. 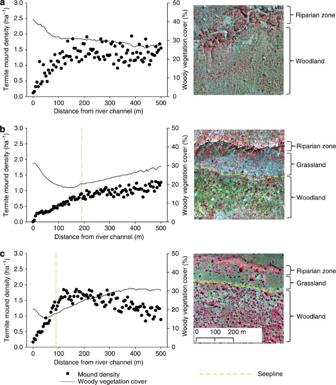Figure 4: Hillslope-scale variation in termite mound and woody vegetation as a function of MAP. Graphs display changes in mound density and woody canopy cover with increasing distance from the river channel. These 2D plots provide an integrated view of the entire 3D landscape in dry (a), intermediate (b) and wet (c) zones. Colour infrared inserts are aerial views of typical hillslopes in each setting. Figure 4: Hillslope-scale variation in termite mound and woody vegetation as a function of MAP. Graphs display changes in mound density and woody canopy cover with increasing distance from the river channel. These 2D plots provide an integrated view of the entire 3D landscape in dry ( a ), intermediate ( b ) and wet ( c ) zones. Colour infrared inserts are aerial views of typical hillslopes in each setting. Full size image The integration of these results provides new insight into the importance of long-term climate in conditioning hillslope-scale hydrology and hence the structure and function of savannas. Minimal hillslope redistribution of clay takes place under relatively dry conditions, hence the seepline is poorly expressed and termite mounds and broad-leafed savanna vegetation are distributed across the entire hillslope ( Fig. 5a ). Intermediate MAP conditions retain clay in valley bottoms and lower slopes, creating broad seasonally saturated grasslands and a well expressed seepline. Outside the riparian corridor, broad-leafed savanna vegetation and termite mounds are restricted to the well-drained sandy crests, but there is sufficient clay present in residual crest soils to support the building of large termite mounds ( Fig. 5b ). Under wetter conditions, long-term chemical weathering of crest soils, and the subsequent removal of clays by colloidal transport, has created a very sandy soil texture that seems to constrain mound building by termites. However, the deep and well-drained crest soils still support tall broad-leafed savanna vegetation and low densities of small termite mounds. Although clays have been mobilized out of the crest and upper slope soils, they are still present in the lower hillslope close to the valley bottom. The seasonally saturated grassland is present but is much narrower than under intermediate MAP conditions, and the seepline is situated further downslope ( Fig. 5c ). Termite mounds are larger and more abundant in the middle of the hillslope where some clay remains, but are absent from the seepline to the riparian zone. Field soil samples taken across this same MAP gradient corroborate this model, as maximum clay retention on the hillslope was found on catenas under intermediate MAP, but dry conditions failed to redistribute as much clay, and wet conditions failed to retain the clay on the upper and middle hillslope sections following production [20] , [21] . 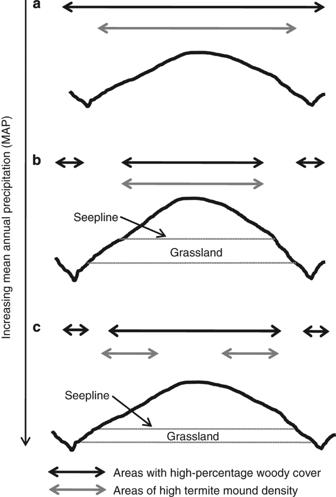Figure 5: Schematic conceptualization of savanna hillslope structure across a mean annual precipitation (MAP) gradient. (a) Minimal hillslope redistribution of clay takes place under drier conditions; hence, a dominant seepline is not present and termite mounds and broad-leafed vegetation are distributed across the entire hillslope. (b) Clay is retained in valley bottoms under intermediate MAP, creating a broad saturated grassland and a prominent seepline. Broad-leafed woody vegetation and termite mounds are restricted to the well-drained sandy crests. (c) Under wetter MAP, the hillslope crests are too sandy to support mound building by termites, but the deep soils still support tall broad-leafed woody vegetation. Clay is still present in the valley bottoms and lower slopes, where termite mounds are larger and more abundant. The saturated grassland is narrower than that under intermediate MAP, and the seepline is situated further downslope. Figure 5: Schematic conceptualization of savanna hillslope structure across a mean annual precipitation (MAP) gradient. ( a ) Minimal hillslope redistribution of clay takes place under drier conditions; hence, a dominant seepline is not present and termite mounds and broad-leafed vegetation are distributed across the entire hillslope. ( b ) Clay is retained in valley bottoms under intermediate MAP, creating a broad saturated grassland and a prominent seepline. Broad-leafed woody vegetation and termite mounds are restricted to the well-drained sandy crests. ( c ) Under wetter MAP, the hillslope crests are too sandy to support mound building by termites, but the deep soils still support tall broad-leafed woody vegetation. Clay is still present in the valley bottoms and lower slopes, where termite mounds are larger and more abundant. The saturated grassland is narrower than that under intermediate MAP, and the seepline is situated further downslope. Full size image The hillslope-scale distribution of vegetation and termite mounds in African savannas is largely determined by long-term climate controls on hydrologic and edaphic properties of catenas. Future shifts in effective moisture will drive a series of ecological responses determined in part by the nature of the catena properties themselves. Current climate models predict a warmer future for most African savannas (SRES scenario A1B) [22] , which, in combination with increased CO 2 fertilization, is likely to facilitate the spread of woody vegetation [23] , [24] . Warming, however, is expected to increase the spatial variability of precipitation [25] , and different savanna regions may become either wetter or drier [22] . In areas with strong catena expression, wetter futures may preclude the spread of woody vegetation into catena grasslands, despite elevated temperatures and CO 2 levels, by increasing the extent and duration of saturated conditions in bottom to midslope positions. However, if these regions become drier, decreased wetting of seasonally saturated zones will promote the spread of woody vegetation into catena grasslands. The mechanisms underlying woody encroachment are therefore not simply physiological responses to elevated temperatures and CO 2 levels but also involve complex hydrological interactions at the hillslope scale. Spatially explicit understanding of hillslope hydrological responses to climatic scenarios will enhance future climate and vegetation modelling efforts. Airborne remote sensing and data collection We operated the CAO [17] over 50,000 ha of savanna in the Kruger National Park, South Africa, in April/May 2008. The CAO integrates high-fidelity imaging spectrometers (HiFIS) with waveform LiDAR sensors for regional-scale ecological research. The CAO combines three major instrument subsystems into a single airborne package: (i) HiFIS; (ii) Waveform LiDAR scanner; and (iii) Global Positioning System-Inertial Measurement Unit (GPS-IMU). The CAO HiFIS subsystem provides spectroscopic images of the land surface. The CAO-Alpha configuration uses a pushbroom imaging array with 1,500 cross-track pixels, and sampling across the 367–1,058 nm range at up to 2.4 nm spectral resolution. The spectrometer subsystem is fully integrated with the LiDAR subsystem having an adjustable laser pulse repetition rate of up to 100 kHz [17] . The GPS-IMU subsystem provides 3D positioning and attitude data for the sensor package onboard the aircraft, allowing for highly precise and accurate projection of HiFIS and LiDAR observations on the ground [17] . The CAO-Alpha configuration provides coaligned HiFIS and LiDAR data at spatial resolutions of 0.4–1.12 m, depending on the aircraft altitude above ground. For this study, the CAO was operated at 2,000 m above ground level, providing data at 1.12 m resolution. All data collection flights were conducted within 3 h of solar noon. Data processing The CAO uses in-flight and postflight data integration approaches to precisely match HiFIS and LiDAR data in 3D space. The in-flight step is achieved by providing a common mount with measured offsets between instrument optical centres, as well as time-stamping of spectral and LiDAR data collection streams with shared position and trajectory data. The LiDAR has a custom-designed laser beam divergence to precisely match the field-of-view of the CAO-Alpha spectrometer. The GPS-IMU data form the common link for the detailed ray tracing of the photons between aircraft sensors and the ground. The GPS-IMU data are combined with the laser ranging data to determine the 3D location of the laser returns. From the laser 'point cloud' data, a physical model is used to estimate top-of-canopy and ground surfaces (digital elevation models; DEMs) using the REALM (Optech) and Terrascan/Terramatch (Terrasolid) software packages. Vegetation height is then estimated by finding the difference between the top-of-canopy and ground surface DEMs [26] , [27] . DEMs derived from LiDAR were analysed in an object-based manner (Definiens Developer, Definiens) to extract termite mound spatial locations and dimensions. Image segmentation was weighted towards changes in slope, and the classification hierarchy considered both the relative difference in elevation between neighbouring objects and image object shape. Data analyses The CAO vegetation data products were field validated in 2008 [28] . Termite mound height estimation from LiDAR was ground validated in April 2009 ( r 2 =0.84, P <0.01, n =150). Woody vegetation and termite mound properties were used to divide the precipitation gradient into three core zones with minimal internal variation for analysis purposes. These zones also correspond to dominant woody vegetation types: 'dry' Colophospermum mopane and Combretum apiculatum savanna; 'intermediate' Combretum apiculatum and Combretum collinum savanna; and 'wet' Terminalia sericea and Combretum collinum savanna. The dominant mound-building termites in this region belong to the Macrotermes . The smallest spatial unit for a zone was 10,000 ha. Size–class distributions of mounds and woody canopy height were compared across the three MAP zones with the Kolmogorov–Smirnov test. Data were randomly subsampled to provide equal sample sizes for comparison ( n =5,000 for mounds; n =10,000 for woody canopy). Changes in termite mound density and woody vegetation cover with distance from river were calculated for the entire 3D landscape and vegetation data set in each MAP zone. The entire hillsope, along the full longitudinal profile of each river, of each stream order, was accessed in 5 m intervals of increasing distance from the river channel. This approach provided integrated 2D plots of variation in woody cover and mound density for the entire landscape within a particular zone. The ecological relevance of the termite mound boundary on vegetation structure was explored through randomly distributed quadrats that were perpendicularly aligned along the downslope extent of termite mound distribution (nonriparian), within each MAP zone. The mean percentage woody cover on the upslope and downslope side of the termite mound boundary was compared with the paired t -test ( n =100, 100 m×200 m quadrats). All statistical procedures were conducted in the R language and environment [29] . How to cite this article: Levick, S.R. et al . Regional insight into savanna hydrogeomorphology from termite mounds. Nat. Commun. 1:65 doi: 10.1038/ncomms1066 (2010).